Correlated motions are a fundamental property of β-sheets Correlated motions in proteins can mediate fundamental biochemical processes such as signal transduction and allostery. The mechanisms that underlie these processes remain largely unknown due mainly to limitations in their direct detection. Here, based on a detailed analysis of protein structures deposited in the protein data bank, as well as on state-of-the art molecular simulations, we provide general evidence for the transfer of structural information by correlated backbone motions, mediated by hydrogen bonds, across β-sheets. We also show that the observed local and long-range correlated motions are mediated by the collective motions of β-sheets and investigate their role in large-scale conformational changes. Correlated motions represent a fundamental property of β-sheets that contributes to protein function. Despite considerable efforts by structural laboratories and the capacity to run long molecular dynamics (MD) simulations, there are still major gaps in our understanding of protein structure and function. Proteins perform the majority of tasks in living cells and integrate signals and functions to produce the controlled responses required for life. While carrying out their functions, proteins undergo changes in conformation as they absorb and dissipate energy, thereby helping to drive reactions and overcome energetic barriers. An obvious and intuitive mechanism to harness the flexibility of proteins is through correlated motions, which can render the flexibility productive in terms of biological function. For allosteric transitions between tense and relaxed states, as well as for enzymes, structure-wide collective changes, often spanning long distances, have been proposed to propagate via pathways that reduce the free energy barriers between such states [1] . The existence of channels of correlated motions is implicitly required as the inter-atomic interactions that govern them decay rapidly with distance [2] . While the mechanisms that cause these behaviours are still largely unknown, recent progress has been made in the study of the allostery of enzymes that contain a central β-sheet, where weakly correlated motions link interaction sites [3] , [4] and store energy for preparation for binding and catalysis [5] . Current views of allostery suggest that correlated motions occur in all proteins [4] , [6] . While for energy storage within localized modes of nonlinear origin, known as discrete breathers, there is a requirement for weak coupling between adjacent peptide planes [5] , [7] . Given the importance of these phenomena, much work has been directed to determining the degree of correlation between the motions of distal sites in the conformational dynamics of proteins [8] . Previous studies focused mainly on the investigation, using theoretical methods, of correlations in the movements of neighbouring residues. Although much of the emphasis was on correlations in the motions of the protein backbone, theoretical as well as experimental observations suggest that side chains can also play important roles in propagating conformational changes over long distances [9] , [10] , [11] , [12] . Recently, there has been significant progress in the analysis of correlated motions by using nuclear magnetic resonance (NMR) spectroscopy [13] , [14] , [15] , [16] and indirect experimental methods such as double-mutant cycles [17] . In a complementary fashion, theoretical methods have also provided insights into the mechanistic details of how inter-residue interactions can lead to correlated motions spanning long distances [18] . Finally, hybrid experimental/computational approaches have also been used to study this phenomenon [19] , [20] , [21] , [22] , [23] . Here we use a database of high-resolution protein crystal structures to determine the fundamental correlated backbone motions occurring in β-sheets. Our results indicate that the motions of the β-strands are coupled by the hydrogen bonding network that stabilizes the sheet, and that this can lead to channels of communication that are perpendicular to the strands. Using molecular simulations, we observe equivalent correlated motions in β-sheet-rich proteins and show that these are associated both with their collective equilibrium fluctuations and with structural transitions between different functional states. The results show that backbone-correlated motions are a fundamental property of β-sheets and that they can be of functional relevance. Extraction of β-sheet motifs from the protein data bank To determine whether backbone correlations are a fundamental property of β-sheets, we compiled a large data set of non-homologous X-ray crystal structures of β-sheet-containing proteins from the protein data bank (PDB). A minimal β-sheet motif, consisting of three neighbouring strands in an antiparallel sheet and defined by the dihedral angles ( φ , ψ and ω ) of two consecutive residues in each strand ( Fig. 1a ), was extracted from the structures. The final ensemble of 18,548 such motifs represents the range of conformations accessible to antiparallel β-sheets at equilibrium and, accordingly, can be used to study the fundamental motions of this element of secondary structure. 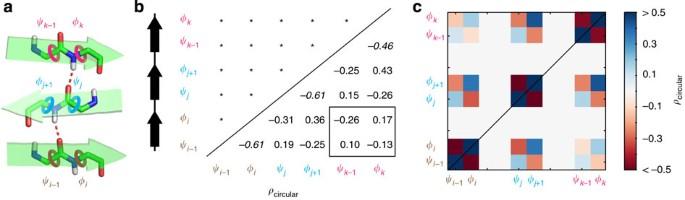Figure 1: β-sheet ensemble correlations observed within and between the strands. The values of the dihedral angle correlation coefficients (ρ) are below the diagonal, and thePvalues for the correlations are given above the diagonal for the β-sheet motif (a). *Correlations were determined to be significantly different from zero to the levelP<0.00001. The 95% confidence interval is ~±0.02 for all correlations. The structure of the β-sheet motif and the associated dihedral angles of the strands are indicated and labelledi,jandkfor the three different strands (b), where residuesi,jandkare opposite one another, as are residuesi−1,j+1 andk−1. The long-range correlations between strandsiandkare highlighted with a box, while the crankshaft correlations are highlighted with italics. A graphical summary (c) of the correlations is shown for comparison withFig. 2. The ensemble was analysed by calculating the circular variance ( Supplementary Table 1 ), the residue bias ( Supplementary Fig. 1 ) and the circular correlation coefficients between the φ and ψ dihedral angles of residues in the β-sheet motif ( Fig. 1b ). Figure 1: β-sheet ensemble correlations observed within and between the strands. The values of the dihedral angle correlation coefficients ( ρ ) are below the diagonal, and the P values for the correlations are given above the diagonal for the β-sheet motif ( a ). *Correlations were determined to be significantly different from zero to the level P <0.00001. The 95% confidence interval is ~±0.02 for all correlations. The structure of the β-sheet motif and the associated dihedral angles of the strands are indicated and labelled i , j and k for the three different strands ( b ), where residues i , j and k are opposite one another, as are residues i −1, j +1 and k −1. The long-range correlations between strands i and k are highlighted with a box, while the crankshaft correlations are highlighted with italics. A graphical summary ( c ) of the correlations is shown for comparison with Fig. 2 . Full size image Characterization of the local correlated motions To determine the strength of all potential correlations, we calculated the circular correlation coefficients ( ρ ) of pairs of dihedral angles. In Fig. 1b , we provide a summary of the correlation analysis, where the crankshaft motion, a rotation of the peptide plane about the C α i −1 –C α i axis that leads to the anti-correlation of ψ i −1 and φ i often observed in MD simulations, is shown in italics [24] . The crankshaft motion is equivalent to that put forward in the one-dimensional Gaussian axial fluctuation model (1D-GAF) of the protein backbone and to the γ motion of the related 3D-GAF motional model, the amplitudes of which have been extensively studied by NMR spectroscopy [20] , [21] , [25] , [26] , [27] . The anti-correlation is due to the rigidity of the peptide plane, which couples the motion of the dihedral angle ψ i −1 with that of φ i while preserving the structure of the strand. In the non-homologous X-ray β-sheet ensemble, we observed that the crankshaft motion leads to an average correlation of ρ ≈−0.6 ( P <0.00001) and can therefore propagate motions between sequential residues. We also observed, as shown in Fig. 1b , correlations in the torsion angles of residues in neighbouring strands, such as a strong correlation of φ and ψ of residues connected by hydrogen bonds. This correlation was also observed in a high-quality conformational ensemble termed ERNST (ensemble refinement for native proteins using a single alignment tensor) that was determined for the small α/β protein ubiquitin by restraining MD simulations with a large set of residual dipolar couplings measured using NMR. This correlation, which we termed β-lever, is caused by concerted crankshaft motions of peptide planes of neighbouring strands in a manner that preserves the inter-strand hydrogen bonds that stabilize the β-sheet [21] . The correlation is stronger between the φ torsion angle of residues in neighbouring strands, with ρ ≈0.4 ( P <0.00001), than between the corresponding ψ torsions, with ρ ≈0.2 ( P <0.00001); the correlations that are combinations of φ and ψ have an intermediate strength, with ρ ≈−0.3 ( P <0.00001). Characterization of the long-range correlated motions As shown in Fig. 1b , long-range correlations were also observed between the first ( i ) and third ( k ) strands. The degree of coupling between these two distal sites is small (| ρ |≈0.1), but the correlations are statistically significant ( P <0.00001) and agree with those observed in the conformational ensemble determined for ubiquitin from NMR data [21] . Figure 1c presents a graphical summary of the correlations observed in the X-ray β-sheet ensemble where the checkerboard pattern, caused by combinations of crankshaft and β-lever motions mediated by relatively rigid hydrogen bonded peptide planes, is distinctive of the correlations occurring in β-sheets. This analysis is based on an X-ray β-sheet ensemble containing non-homologous proteins and can therefore be used to analyse the properties that are common to all residue types, such as the backbone and the hydrogen bonds, but not those that are specific to certain protein structures or folds. To investigate the influence of fold-specific structural heterogeneity, we compared the results obtained with this X-ray β-sheet ensemble to those obtained for ensembles representing the structural heterogeneity of six different folds. The average correlation map for each of these ensembles considered was remarkably similar to that obtained for the non-homologous ensemble, but significant variations between motifs within the folds were observed ( Supplementary Fig. 2 ). Site-specific enhancements, and in some cases marginal distance dependence of the correlation strength, were observed for the six protein folds considered, supporting the hypothesis that the backbone correlations observed in the non-homologous ensemble can play a role in allostery when they are strengthened by those specific to the protein fold. Correlations in a model β-sheet The most relevant motions in β-sheets are twisting and bending with respect to an in-plane axis perpendicular to the β-strands ( Fig. 2 ). Emberly et al. [28] observed from a principal component analysis (PCA) that twisting and bending were the first and second functional deformation modes of isolated β-sheets, together accounting for half the atomic variance (Å 2 ). It is also known that normal mode analysis (NMA) predicts very similar motions to those observed in MD simulations [18] , [29] , [30] , [31] , [32] and, accordingly, similar patterns of correlations. The correlations observed in the non-homologous X-ray β-sheet ensemble, summarized in Fig. 1c , were comparable to those observed in ensembles generated by using all-atom NMA in an elastic network model (ENM) and in the CHARMM27 force field, which are known to give similar results [33] , [34] , [35] , for a channel of six peptide planes in a model β-sheet. For both methods, the signs of the local and long-range correlations of the channel were found to be equivalent to those observed in the non-homologous X-ray β-sheet ensemble ( Fig. 2a,b and Supplementary Figs 3 and 4 ). Visual inspection of the elastic normal modes of the isolated β-sheet motif revealed that modes 1 and 2 correspond to sheet bending and twisting, represented in Fig. 2c,d , consistent with earlier reports. The correlation coefficients from the NMA of individual modes can be quite high (| ρ |≈0.9) and do not decrease as a function of distance because the displacement along the elastic normal modes produces the pure concerted motions. This is in contrast to the non-homologous X-ray β-sheet ensemble, where a distance dependence of the correlation magnitude was observed. We note, however, that simultaneous displacements along multiple modes would lead to a distance dependence as would averaging of correlations over multiple motifs, as observed in ensembles representing the structural variability of specific folds ( Supplementary Fig. 2 ). An analysis of the low-frequency modes (3–10) shows that the correlations were mostly consistent with the non-homologous β-sheet ensemble; however, there are regions where there is disagreement ( Supplementary Figs 3 and 4 ) due to contributions of overtones of the fundamental mode frequencies. Despite the disagreement in some regions of the β-sheet, regions of agreement were found in many of the first 10 normal modes, as identified by the alternating checkerboard pattern of positive and negative dihedral correlations. Thus, both sheet twisting and bending were observed to dominate the low-frequency elastic modes of motions in the model β-sheet. 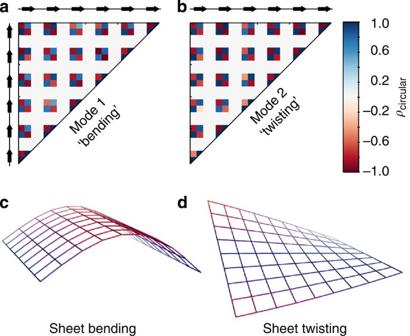Figure 2: Correlations caused by primary modes of motion in β-sheets. Graphical summaries of the correlations coefficients (ρ), for comparison withFig. 1, are shown for the first two all-atom elastic normal modes for six central strands of the model β-sheet structure that best agreed with the correlations observed for the β-sheets ensemble (a,b). The mode 1 corresponds to the bending mode (c) and mode 2 corresponds to the twisting mode (d). Figure 2: Correlations caused by primary modes of motion in β-sheets. Graphical summaries of the correlations coefficients ( ρ ), for comparison with Fig. 1 , are shown for the first two all-atom elastic normal modes for six central strands of the model β-sheet structure that best agreed with the correlations observed for the β-sheets ensemble ( a , b ). The mode 1 corresponds to the bending mode ( c ) and mode 2 corresponds to the twisting mode ( d ). Full size image Correlations in MD simulations of β-sheet-rich proteins The β-sheet model and the non-homologous X-ray β-sheet ensemble exclude the variability between β-sheets in distinct proteins. We focus now on determining whether the correlations can be detected in MD simulations of a heterogeneous set of 24 β-sheet-rich proteins. To remove the fluctuations arising from high-frequency vibrations, we performed PCA of the MD trajectories. The first PCA components describe the large-scale collective motions of a structure, which are of functional relevance and are also similar to the normal modes from ENMs. We used Brownian dynamics (BD) [36] , [37] to populate ensembles along the first PCA component and obtained the results presented in Fig. 3 , which highlights the regions in which long-range correlations are observed in 12 selected proteins. The first principal component of MD trajectories is known to be the most anharmonic one and is often associated with biologically relevant motions [38] , [39] . We note that using the first five PCA components gives the same result as using the first normal modes because the first modes concentrate most of the structural variance ( Supplementary Table 2 ). Furthermore, the ensembles of homologous proteins described above similarly sample the first PCA component of the MD simulations ( Supplementary Fig. 2 ). To quantify the agreement of the correlations in an individual motif with those calculated from the X-ray ensemble, we calculated a motif score, which is a count of the number of pairs of dihedral angles with correlations of the same sign as in the homologous X-ray ensemble and takes values between zero and 15, with a value of 15 indicating perfect agreement between the checkerboard pattern observed for the X-ray ensemble. Our results indicate (red regions of the structures with motif scores >10 in Fig. 3 ) that the motion along the first principal component of MD trajectories does indeed give rise to the checkerboard pattern of correlations described in Fig. 1c . 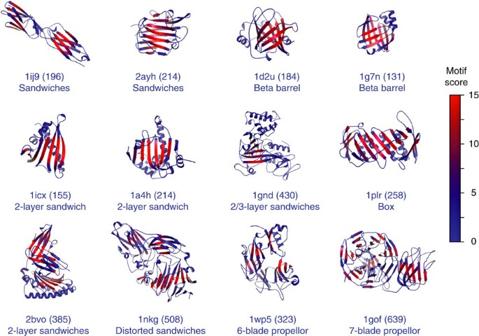Figure 3: β-sheet-rich proteins with minimal motifs that show correlations. The structures are coloured according to the motif score, which has a maximum value of 15 and indicates that the β-sheets move in a correlated way as predicted from the PDB and the all-atom NMA analysis. The probability of observing the red highlighted regions that correspond to values >10 and have a random probability of <0.06 under independence. The correlations were extracted from coarse-grained BD simulations that were generated using the first PCA mode from all-atom MD simulations taken from the MoDEL project39. The backbone coordinates were then rebuilt from the coarse-grained Brownian trajectories before calculating the circular correlation coefficients as previously discussed. We note that the results are invariant if more PCA modes are used in the BD (data not shown), similar trends are observed if NMA modes are used instead of the PCA modes. Figure 3: β-sheet-rich proteins with minimal motifs that show correlations. The structures are coloured according to the motif score, which has a maximum value of 15 and indicates that the β-sheets move in a correlated way as predicted from the PDB and the all-atom NMA analysis. The probability of observing the red highlighted regions that correspond to values >10 and have a random probability of <0.06 under independence. The correlations were extracted from coarse-grained BD simulations that were generated using the first PCA mode from all-atom MD simulations taken from the MoDEL project [39] . The backbone coordinates were then rebuilt from the coarse-grained Brownian trajectories before calculating the circular correlation coefficients as previously discussed. We note that the results are invariant if more PCA modes are used in the BD (data not shown), similar trends are observed if NMA modes are used instead of the PCA modes. Full size image Correlations in functional transitions of β-sheet proteins To investigate whether functional structural transitions occur via changes that invoke β-sheet long-range correlated motions, we studied five proteins for which two distinct conformers have been reported in the PDB ( Supplementary Table 3 ). The smallest ones (1szv, 1s2h) are single domains with a central β-motif, whereas the rest are multi-domain proteins (1ram, 3dap, 1rkm). To gain a detailed insight into the role of β-sheets in these structural transitions, we used unrestrained MD simulations to determine the stiffness of the pure bending and twisting motions and evaluated the approximate deformation energies for the structural transitions pathways generated by BD. The β-sheet-rich regions of all five proteins produced the characteristic checkerboard pattern of long-range correlations as they sampled their structural transitions ( Supplementary Fig. 5 ). These conformational changes result in significant local deformations of the β-sheets between 0.5 and 2.5 Å and are associated with binding to other proteins, to large ligands or to small molecules, which triggers global structural changes ( Supplementary Table 3 ). In all cases, the first 10 PCA modes from the unrestrained MD simulations described well the experimentally observed structural transition with overlaps of ~80%. We focused our analysis on the main β-sheet present in each structure, which was the largest β-sheet present in the structure and which also corresponded to the β-sheet containing the highest number of β-motifs displaying correlations. For each β-sheet, we measured the bending and twisting angles of the β-sheet both along the BD transition pathways and unbiased MD simulations ( Supplementary Table 3 ). In all cases, the structural transitions were related to significant (2–10°) bending or twisting of the β-sheet ( Fig. 4 ). The stiffness constant for motif bending was on the order of 0.5–1 k B T Å −2 , while the stiffness constant for motif twisting was as high as 3 k B T Å −2 . We also estimated the elastic energy required for the correlated bending and twisting deformation of the β-sheet during the conformational transition, finding that energies in the range of 5–15 k B T or ~0.02 kcal mol −1 residue −1 could be stored and potentially exchanged. 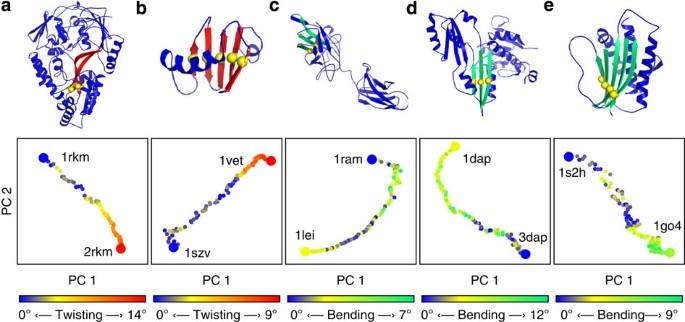Figure 4: Correlated motions along transition pathways. β-sheet-rich regions of the structures are coloured red or green to indicate either dominant twisting (a,b) or dominant bending (c,d,e), respectively. The overlapping channels of motifs associated with the principal motif are shown in yellow. Transition pathways projected onto the first two PCA components from unrestrained MD simulations are coloured with red or green to indicate the dominant twisting or bending, respectively, during the structural transition. The colour gradient indicates the change in degrees of the twist or bend from the start of the transition pathway. The two experimentally determined structures of the transition pathways are shown with larger point sizes. Figure 4: Correlated motions along transition pathways. β-sheet-rich regions of the structures are coloured red or green to indicate either dominant twisting ( a , b ) or dominant bending ( c , d , e ), respectively. The overlapping channels of motifs associated with the principal motif are shown in yellow. Transition pathways projected onto the first two PCA components from unrestrained MD simulations are coloured with red or green to indicate the dominant twisting or bending, respectively, during the structural transition. The colour gradient indicates the change in degrees of the twist or bend from the start of the transition pathway. The two experimentally determined structures of the transition pathways are shown with larger point sizes. Full size image We observed the crankshaft motion to be the main motion occurring in the non-homologous X-ray ensemble. The strength of the backbone correlation associated with this motion ( ρ ≈−0.6) was found to be similar to that derived from conformational ensembles determined with [20] and without [8] restraints derived from experimental NMR parameters. This ensemble accurately reproduced the residual dipolar couplings, as well as other experimental NMR parameters that were not used to bias the simulations, and its analysis revealed the presence of long-range correlated motions across the β-sheet of ubiquitin. The strength of the crankshaft correlation in the ubiquitin ensemble was found to be −0.7±0.2 in β-strands, which is comparable to the value of −0.6 obtained in the non-homologous X-ray ensemble presented here [21] . The correlations between the backbone torsion angles of residues in neighbouring strands of β–sheets were also found to be equivalent to those observed in ubiquitin [21] . For the ERNST ensemble, the β-lever gave an average correlation of ρ ≈−0.3, in agreement with the results reported here, which range between −0.2 and −0.4 [21] , [27] . The weaker correlation observed for motions involving ψ angles may be due to the presence of an additional and previously described correlation between ω and ψ , which was attributed to electronic interactions of the backbone [40] , and which results in a slight decoupling of the changes in ψ from the motions of the hydrogen bonded peptide planes. The attenuated correlations associated with ψ may also in part be due to bifurcated hydrogen bonds in which the CO group of a residue in one strand is hydrogen bonded to both the NH group and to the C α H α group of the preceding residue in the opposite strand [41] . The correlations associated with the β-lever are caused by the geometrical restraints of the approximately fixed C α positions, the planarity of the peptide bond and the conserved nature of hydrogen bonding distances and angles. The correlations of φ with ψ in opposing strands are of negative sign while those of φ with φ and ψ with ψ are instead positive because the rotation of a peptide plane in the clockwise direction around the C α i −1 –C α i axis causes an equivalent clockwise rotation of the peptide plane in the neighbouring strand [19] , [20] , [21] . We observe circular variances, which range between zero and one and where low values indicate tight clustering around the mean, of 0.038 for φ and 0.029 for ψ . These are within the range observed in the ERNST ubiquitin ensemble (0.031±0.017 and 0.021±0.014, respectively) and correspond to s.d. of 16.0 and 13.9°. The lower variance of ψ is also consistent with the existence of bifurcated hydrogen bonds in antiparallel β-sheets [41] . This observation confirms that the β-sheet undergoes dynamic changes without compromising the stability of the structure and that the network of weak correlations between neighbouring strands is due to the combination of the crankshaft and β-lever motions. Our results also show that long-range correlations between non-neighbouring strands exist, and lead to collective changes in β-sheets. The long-range coupling between the first and third strands appears to be additive, as the product of the two β-lever correlations φ i / φ j and φ j / φ k (0.36*0.43=0.15) is approximately equivalent to the strength of the long-range correlation observed between the non-neighbouring strand dihedrals ( φ j /φ k ) 0.17±0.02. We note that this equivalence is for the pathway proceeding through φ and does not hold for a potential pathway through ψ j involving the correlations φ i / ψ j and ψ j / φ k (0.31*0.26=0.08). Thus, as was observed for the β-lever motion, the long-range correlations are reduced when measured between ψ angle rotations. We conclude from the observation of long-range correlations in the non-homologous X-ray β-sheet ensemble that these correlations are a consequence of the hydrogen bonding network, as this is the only remaining property that can link the strands across the β-sheet motif. The general occurrence of correlated motions in the X-ray β-sheet ensemble underlies the cooperative nature of this secondary structure element and the large fluctuations of the dihedral angles indicate that these structures can be highly dynamic. While the average correlations in the motif are weak, we observed from the homologous structure ensembles that fold-specific structural heterogeneity leads to correlations in certain regions of the structure to become much stronger. Thus, additional factors influence the correlations in a sequence and fold-specific manner to enhance or diminish the correlations. Side chains are likely candidates as an additional factor. NMR studies of side chain dynamics [42] and double-mutant cycles [17] have shown that side chains can produce non-additive interactions that can be coupled to backbone motions [43] . The observations of equivalent patterns of backbone correlations in both the normal modes of the model β-sheet and the large set of BD ensembles of β-sheet-rich proteins indicate that local and long-range correlations participate in the large-scale motions occurring in β-sheet-containing proteins. While in a complementary way, the BD transition pathways reveal how the series of weak but long-range inter-strand correlations in the β-motifs create channels for the propagation of structural information from one end in the β-sheet to the other one, spanning distances up to 20 Å, and thus transmitting changes between distant regions through global conformational changes. The observed stiffness values and the eigenvalue variances are in qualitative agreement with the work of Emberly et al. [28] as do the elastic energies required for the correlated bending and twisting of the β-sheet during the conformational transitions [44] , [45] . This suggests that twisting and bending may be carefully encoded in the structure of β-sheet-rich proteins to store and potentially exchange energy to perform their biological roles. One illustrative example is the large-scale conformational change found in the periplasmic binding protein OppA ( Fig. 4 ), which occurs between open and closed states and where transitions between these states appear to be concomitant with correlated motions of the β-sheet. The ligated (1rkm) and unligated (2rkm) forms of OppA are related by a rigid-body rotation of domains I and II with respect to domain III. The hinge region that mediates the rotation is composed of two β-sheet segments where correlated changes in the backbone dihedral angles ϕ and ψ are responsible for the structural transition. The twisting motion of the β-sheet embedded in the inter-domain interface mediates the conformational change. These examples of functional transitions show that the correlations that exist within correlated motions may define routes for conformational transitions, and can act as a mechanism to propagate information throughout the protein backbone. We have shown in a force field-independent fashion that the fluctuations of backbone dihedrals in the β-sheet of proteins are correlated. We have also shown that these correlations are related to the functional deformation modes of this secondary structure element, derived from the geometry of the β-sheets and from the requirement of maintaining inter-strand hydrogen bonds. Our results have established that these β-sheet-correlated motions provide mechanistic pathways that can allow functional transitions between distal sites. They in addition indicate that the local and long-range correlated motions described here can contribute to protein function. Generation of the β-sheet ensembles The non-homologous X-ray β-sheet ensemble was generated by selecting from the PDB protein-only structures with a sequence longer than 50 residues and a minimum resolution of 2.5 Å. In addition, sequence homologues were removed with an identity cutoff of 95%. This gave a list of 16,179 files containing 17,216 unique structures as determined by the homology criteria. A list of the structures is available from the authors on request. The structure database was then further curated to remove atoms with B-factors >50, ensuring that undefined coordinates were removed from the structures before generation of the β-sheet ensemble. The residue secondary structure was determined using the DSSP selection criteria. For all residues in β-sheets as determined using DSSP [46] , we tested whether a given peptide plane ( j and j +1 ) fulfilled the criteria of the β-sheet motif. Only complete β-sheet motifs were added to the β-sheet ensemble. The residue and dihedral indexing defines three antiparallel strands indicated in Fig. 1b and labelled i , j and k for the three different strands, where residues i , j and k are opposite one another, as are residues i −1, j +1 and k −1. Eight criteria were used for selection of the strict motif for a given peptide plane ( j and j +1 ): (1) residues j and j +1 must have β-sheet secondary structure as determined by DSSP; (2) residue j must be a hydrogen bond acceptor to residue i ; (3) residue j +1 must be a hydrogen bond donor to residue k −1 ; (4) residues i and k must be in a β-sheet and be opposite residue j ; (5) residues i −1 and k −1 must have β-sheet secondary structure and be opposite residue j +1 ; (6) flanking residues i +1 , i −2 , j +2 , j −1 , k +1 and k −2 must have β-sheet secondary structure; (7) φ and ψ angles of all residues including the flanking residues must be in the correct Ramachandran quadrant; φ ≤0° and ψ ≥45° or ψ ≤−135°; (8) the motif or flanking residues (see 6 above) must not include the residue types glycine or proline. These selection criteria gave rise to the β-sheet ensemble containing 18,548 β-sheet motifs. The circular variances of the dihedral angles are given in Supplementary Table 1 . To ensure that a residue type bias was not producing the observed correlations, we present Supplementary fig. 1 , where we show that the amino-acid distribution at all positions in the β-sheet motif are the same. The minimal motif was selected by excluding criteria 6 from the selection. The homologous ensembles ( Supplementary Fig. 2 ) were generated by selecting sequence homologous NMR ensembles and X-ray structures to 1cbs (78 structures), 1mvg (60 structures), 2axf (80 structures), 1rkm (32 structures), 1s2h (33 structures) and 1szv (56 structures). The minimal motifs were extracted from each structure and then analysed separately. Finally, the motifs were combined and analysed together to obtain the correlations for the average motif of each structure. Examples of the highest- and lowest-scoring motifs are shown in Supplementary Fig. 2 . Circular statistics and correlations The circular mean, variance and correlation coefficients were used as defined by Jammalamadaka and Sengupta [47] . The mean angle is then given by the quadrant-specific inverse of the tangent as While the circular variance (CV) is defined as; The correlation coefficients were calculated using the method put forward by Jammalamadaka and Sengupta [47] , which is appropriate when both data come from circular distributions. The circular correlation coefficient is defined as The correlations were calculated for all the combinations of φ and ψ torsion angles in the β-sheet motif. The φ and ψ torsion angles were defined by the heavy atoms in the backbone of the protein. For the correlation matrices, we present only the significant correlations as determined from random permutation approach. The P values were obtained by comparing the observed circular correlation coefficient with those obtained after randomly permuting the values of the torsion angles. One hundred thousand permutations were used. Generation of the normal model ensembles A synthetic all-atom model β-sheet consisting of 14 strands was generated by repeatedly excising and aligning strands from the structure of the sucrose-specific porin ScrY from Salmonella typhimurium [48] . The residues that were extracted were 290–294, 309–313, 337–341, 357–361, 373–377 and 397–401 (strands A–F). Three of these sheets were joined together by aligning strands A and B with the last two strands (E and F) of the three sheets. The terminal strands (A and F) were then removed from the overlapping regions to generate a contiguous sheet (A,B,C,D,E,B,C,D,E,B,C,D,E,F). The residues were all mutated to alanine and the missing atoms built. The model β-sheet structure was then minimized using the CHARMM27 force field with the generalized Born with simple switching (GBSW) implicit solvent for 100 steps [49] . The minimized coordinates were then submitted to the ENM server elNémo to determine the elastic normal modes of the system and to obtain displacements of the modes for the model β-sheet [50] . The elastic normal modes were calculated using the a distance cutoff of 8 Å for the identification of elastic interactions and a value of 1 for NRBL. For each of the first 10 modes (1–10), the displacements were then calculated using DQSTEP step=1, DQMIN=−20 and DQMAX=20. The values of DQMIN and DQMAX were lower than the default values, as higher values gave rise to large distortions in the structure. The ensemble of 41 structures was then minimized using the CHARMM27 force field with the GBSW implicit solvent for 100 steps to remove any strain in the structures produced during the generation of the displacements. The correlations in the normal mode ensembles were analysed for a channel of peptide planes connected by hydrogen bonds that ran across the peptide planes by using the same procedure used for the β-sheet motif for the first 20 mode displacements, as these represented right-handed twisting from the starting structure. Graphical summaries of the correlations coefficients for strands four to nine are shown in Fig. 2 and Supplementary fig. 3 . Normal modes and trajectories of mode displacements were additionally calculated from the same structure used in the elastic normal mode calculations using GROMACS with the CHARMM27 force field combined with the OBC (Onufriev, Bashford, Case) implicit solvent model [51] . The structure was thoroughly minimized to reach a minimum before the normal mode analysis was made in GROMACS [52] . The displacement trajectories were minimized before the correlation analysis as for the ENM calculations, and graphical summaries of the correlations coefficients for strands four to nine are shown in Supplementary Fig. 4 . MD simulations and PCA All MD simulations analysed in this paper were extracted from the MoDEL database [39] , a large collection of atomistic trajectories for representative protein folds computed using state-of-the art standard protocols. High-frequency motions from MD simulations were filtered by PCA using pcatool, a development tool for the calibration of NMA calculations against MD and experimental structural ensembles [53] . Generation of the BD ensembles Ensembles were generated for each protein as in Supplementary Table 2 by using a coarse-grained BD simulation for the C α atoms [31] , [36] , [39] . The simulations are biased to sample functional modes, which are either normal modes from ENMs (ENM-NMA) or PCA of MD simulations (MD-PCA). During the BD simulations, the protein was kept at constant temperature using a stochastic bath and the motion for each C α particle ( r i ), was given by a Langevin equation: where the second term represents a dispersive force, accounting for the viscous resistance of the solvent (depending on a friction coefficient γ ), and where ξ i (t) is a Gaussian noise term, which accounts for molecular-thermal collisions with surrounding solvent. The force acting on each C α particle, F i , is computed assuming harmonic potentials for its interactions with the other particles of the system ( j ): Where N is the number of C α particles in the protein, r ij and are the instantaneous and equilibrium distances between each pair of C α ’s ( i and j) , and K ij is the corresponding spring constant defined by the algorithm [31] , where emphasis is made in local contacts to ensure the maintenance of the backbone structure. Note that this algorithm strongly weights nearest-neighbours interactions as the dominant ones. Contacts up to i , i +3 are 10 2 to 10 4 stronger than the rest of the contacts. An additional size-dependent cutoff was used to set long-range contacts near or equal to zero. The algorithm guarantees efficient harmonic sampling along the functional modes, derived from either PCA-MD or ENM-NMA by an additional biasing force [36] . The additional biasing force is derived from eigenvectors/eigenvalues obtained from either PCA of atomistic MD simulations or NMA of ENM potentials. The force is given by: Where e k and λ k are the eigenvectors and eigenvalues defining the perturbation force due to the displacement along the first k mode, and is the force due to the harmonic interactions mimicking the internal covalent and non-covalent forces. The stochastic differential equation 4 is solved as in Carrillo et al. [36] , by using the Verlet algorithm to numerically integrate the velocities from the positions. For simplicity, calculations in Supplementary Table 2 were performed using a restricted set of m =1 or m =5 eigenvectors (similar results were obtained using the first 10 eigenvectors). The backbone coordinates of the resulting 1,000 trajectory frames were then reconstructed using PULCHRA, which optimizes the hydrogen bonding geometry for the backbone atoms [37] . The circular correlation coefficients were then calculated for all the motifs in these structures. The directions of the correlations were then compared with those in the checkerboard pattern that we observed in the PDB ensemble. The motif score represents the number of correlations with the correct sign, and has a maximum value of 15 and a minimum value of 0. The combinatorial probabilities for observing a score >10 is <0.06 under the condition of independence. In Supplementary Table 2 , we list the 24 structures for which we made calculations. Generation of structural transition ensembles We selected five different open/closed protein pairs with displacements > 2 Å r.m.s.d. from the molecular motions’ database [54] . These examples have different sizes (91–517 amino acids) and correspond to a wide variety of macromolecular motions. The structures are relatively large and conform to the quality scores of the standard structure validation program Molprobity [55] . Hydrogen atoms were added to each conformation before checking its structural integrity. Conformational transition pathways were generated using the BD algorithm discussed above together with a dynamic importance sampling algorithm incorporated to guide the simulation towards the target structure, instead of eigenvectors/eigenvalues obtained from ENM-NMA or MD-PCA [56] , [57] . The biasing function for the dynamic importance sampling was the sum of internal distances of the target structure. The resulting frames describing the transition pathways were reconstructed with PULCHRA and analysed for circular correlations (results in Supplementary Table 3 ). The structures are coloured according to the motif score, which has a maximum value of 15 and indicates that the β-sheets move in a correlated way as predicted from the PDB and the PCA as shown in Supplementary Fig. 5 . We observed that the β-sheet regions of these five proteins changed as predicted by the long-range correlations, suggesting a distinct functional role for these correlations in the biological function of these proteins. We illustrate in Supplementary Fig. 6 the results obtained for two typical examples: p14 and NF-κB. We observed that the β-sheet-rich regions of the two domains produced the characteristic checkerboard pattern of the long-range correlations and low-frequency modes (panel c of Supplementary Fig. 6 ). Energy associated with β-sheet bending and twisting For each of the ‘open’ structures in Supplementary Table 3 we calculated the energy associated with the conformational change. We ran unrestrained MD simulations using the standard MoDEL protocols [39] . For the set of five conformational transition pairs, we performed PCA on the unrestrained MD simulations for both the full protein and the isolated primary β-motif present in each. These motifs displayed long-range correlations (see Supplementary Fig. 5 ). The PCA of the entire structure yields a set of functional modes (Full-PCA) that describe the global conformational change, whereas the PCA of the reduced covariance matrix for the isolated β-motif (β-PCA) filters the pure bending and twisting modes that were distributed in the first principal components of the entire protein. We calculated the overlap (O 10 ) of motions from the unrestrained MD simulations with the observed X-ray conformational changes. The similarity between the unrestrained MD simulations and the experimental transition is measured for each PCA mode of the MD simulation as the sum of the m -important deformation modes (the minimum set explaining a given threshold of protein motions, that is, variance), which yields a similarity index ranging from 0 (no similarity in the directions of motion) to 1 (perfect similarity): Where α k is defined as: where Δr= ( R 2 −R 1 )/ ‖ R 2 −R 1 ‖ is the unitary transition vector between the two sets of coordinates, R 1 and R 2 , describing the observed states of the protein and ν k is the k th MD-PCA mode. The eigenvalues of the first and second β-PCA modes are proportional to the bending and twisting constants and scale with the number of strands as reported in Emberly et al. [28] These eigenvalues were used to obtain an estimate of the bending and twisting stiffness of the β-sheets via correlated torsions of the backbone in the nanosecond timescale. Sheet bending (Θ bend ) and twisting (Θ twist ) angles for the primary β-motif present in each structure were calculated for the MD simulations and the conformational transitions (see Supplementary Table 3 ). In the context of functional large-scale structural transitions, the pure bending and twisting modes (the first and second β-PCA modes) are split over several modes involving collective motions. To evaluate the potential energy stored in the correlated deformation of the β-sheets along complete functional transitions, we used Mahalanobis distance for the first 10 modes from the Full-PCA [58] . This metric defines Euclidean distances weighted by the variance of every degree of freedom, which in the principal component orthogonal basis can be written as: where x i is the displacement along individual eigenvectors, λ i stands for the corresponding eigenvalue (in units of distance 2 ) and the sum extends over the space of the first 10 PCA modes ( m =10). The Mahalanobis distance represents the simplest deformation coordinate to drive a transition, assuming a harmonic relationship between displacements from the minimum and energy. Thus, in the harmonic limit, the energy associated with displacements along principal components to reach the target structure can be easily determined from the Mahalanobis distance as: As can be seen in Supplementary Table 3 , the transitions of all five proteins are well described by first 10 PCA modes (with typical overlaps above 0.8), and therefore it is possible to estimate the elastic energy of deformation along the conformational change from the Mahalanobis distance. For a conformational transition between two states, the minimal displacement along individual eigenvectors, x i , corresponds to the projection of the transition vector, Δ R AB , onto each PCA mode i : Where Δ R AB is defined only for the subset of residues belonging to the primary β-sheet motif present in each structure. Projections for each of the transition pathways onto the MD subspace defined by the first two principal components of the Full-PCA are shown in Fig. 4 , accompanied by the change in bending or twisting angle of the primary motif in each for each conformer along the transition pathway. How to cite this article: Fenwick, R. B. et al. Correlated motions are a fundamental property of β-sheets. Nat. Commun. 5:4070 doi: 10.1038/ncomms5070 (2014).